A cortical–spinal prosthesis for targeted limb movement in paralysed primate avatars Motor paralysis is among the most disabling aspects of injury to the central nervous system. Here we develop and test a target-based cortical–spinal neural prosthesis that employs neural activity recorded from premotor neurons to control limb movements in functionally paralysed primate avatars. Given the complexity by which muscle contractions are naturally controlled, we approach the problem of eliciting goal-directed limb movement in paralysed animals by focusing on the intended targets of movement rather than their intermediate trajectories. We then match this information in real-time with spinal cord and muscle stimulation parameters that produce free planar limb movements to those intended target locations. We demonstrate that both the decoded activities of premotor populations and their adaptive responses can be used, after brief training, to effectively direct an avatar’s limb to distinct targets variably displayed on a screen. These findings advance the future possibility of reconstituting targeted limb movement in paralysed subjects. Brain–machine interfaces (BMIs) provide a unique opportunity for restoring volitional movement in subjects suffering motor paralysis. Neurons in many parts of the brain including the primary motor and premotor cortex, for example, have been shown to encode key motor parameters such as motor intent and ongoing movement trajectory [1] , [2] , [3] , [4] , [5] , [6] . In line with these findings, awake-behaving animals can use the activity from a fairly small number of neurons in the motor cortex to control external devices such as a computer cursor on a screen or a mechanical actuator [7] , [8] , [9] , [10] , [11] , [12] , [13] , [14] , [15] , [16] , [17] , [18] , [19] . More recent studies have also demonstrated the possibility of controlling devices such as a robotic arm to produce fluid three-dimensional movements [9] , [11] , [12] , [17] . While these approaches have provided key advancements in artificial motor control, another important goal has been to control the naturalistic movement of one’s own limb. This prospective capability is particularly attractive in that it could eventually limit the need for mechanical devices to generate movement [15] , [20] , [21] . Unlike the control of external devices, however, a distinct problem in attaining limb movement control is that the output of the motor system (for example, the corticospinal tract and its associated afferents) is generally not explicitly known. For example, when controlling a mechanical device or cursor with a BMI, an experimenter can determine which output commands will move the device up or down. In contrast, the exact combination of successive agonistic and antagonistic muscle contractions naturally used to produce limb movement to different targets in space is difficult to explicitly ascertain or reproduce [22] , [23] , [24] , [25] . One approach aimed at addressing this problem has focused on using cortical recordings to determine the ongoing trajectory of intended limb movement [20] . For example, the same muscles that were active during training can be stimulated in sequence to produce muscle contractions that lead to limb movement over a similar trajectory, thus, producing repeated movements to a single object in space. Another approach has also used changes in the activities of individual neurons to direct the contraction force of opposing muscles in order to smoothly move a lever in a line [21] . These approaches have, therefore, provided an important advancement in our ability to mimic the trajectory and velocity of planned movement. However, a fundamental present limitation in these methods is that they are principally aimed at producing movements to a single target at a time or movements within one-dimension. This limitation occurs because the possible combination of distinct muscle contractions significantly increases as the number of possible movement trajectories grows [24] , [25] , especially when considering movement outside 1D or in cases where the limb is not narrowly constrained to follow a single repetitive path. While generating such movements can be quite valuable, another compelling goal is the design of a neural prosthetic that can allow subjects to perform movements in higher dimensional spaces and to more than one repetitive target. Here, we aimed to address this problem from an alternate perspective by focusing on the target of movement itself instead of the intervening ongoing trajectory. We hypothesized that if the intended targets of movement are known, it may be possible to match these with stimulation parameters that elicit limb movements programmed to reach the precise intended targets in space. Specifically, if the planned target of movement can be determined from cortical recordings and if the targets of movement produced by different stimulation sites/parameters can be empirically ascertained, we may be able to elicit limb movement to distinct targets under volitional control. Moreover, this approach would not require an explicit determination of which sequence of muscle contractions or limb kinematics is needed to produce such targeted movement. Towards this end, we develop a real-time cortical–spinal neural prosthesis in monkeys that infers the planned target of movement based on changes in premotor neuronal activity and then matches this information with spinal cord and/or muscle stimulation parameters that elicit movements to the same intended targets on a two-dimensional screen. To test this prosthesis in functionally paralysed animals, we also devise a novel dual-primate paralysis model that eliminates the potential influence of afferent/efferent pathways such as partially preserved movement or proprioceptive feedback in the tested animals. This is particularly important, since proximal movement and proprioceptive feedback, which are lost in paralysis but may be preserved by local nerve block, are strongly represented in the motor cortex [26] , [27] . Moreover, healthy subjects can control a BMI more accurately if provided with such feedback [26] . Finally, we examine two distinct approaches for controlling targeted movements based on either decoded neural population activity or their adaptive response. As an initial proof of concept and to test these two approaches, we focus on producing movements to two possible distinct targets during real-time neural–prosthetic control. Our experiments demonstrate that functionally paralysed primates are able to precisely reach the different displayed targets on a screen by using cortically controlled stimulation-elicited limb movements within a plane. We compare the performance of neural population decoding versus adaptive neural activity for controlling such targeted limb movements, and discuss the potential benefits and drawbacks for using these techniques. Dual-primate avatar model for motor paralysis To test volitional motor control in awake-behaving animals without confound of intact efferent/afferent spinal pathways, we first devised a novel dual-primate motor paralysis model. Here, two adult Rhesus monkeys ( Macaca mulatta ) were separately designated as either a master or an avatar on different sessions. The monkey functioning as the master was responsible for controlling movement based on cortically recorded neural activities, and the other sedated monkey functioned as the avatar and was responsible for generating movement based on distal spinal cord and/or muscle stimulations. Since the sedated avatar was a separate animal from the master and therefore had no physiological connection with the master, the master had no direct afferent or efferent influence on the avatar’s movement and was, therefore, fully paralysed from the functional standpoint ( Fig. 1 ). The two monkeys were interchangeably used as the master or the avatar on alternate sessions, meaning that we effectively tested two masters and two avatars in this study. 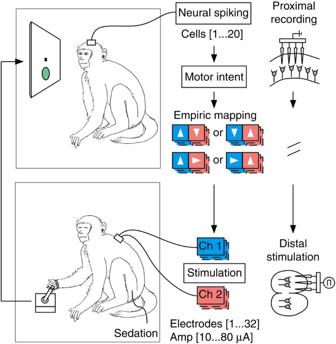Figure 1: Schematic illustration of the dual-primate set-up. The master is displayed on top and the avatar is displayed on the bottom. Note that on decoding-based sessions, the master had a joystick during training that was then disconnected during the real-time neural prosthetic trials. On adaptive-based sessions, no joystick was used at any time. Under ‘empiric mapping’, the arrows indicate the estimated intended target of movement based on neural activity and the colour codes illustrate the corresponding stimulator channel used to elicit limb movement in the animal. The left versus right pairings indicate the two possible mappings to movement to each of the targets for the first and second avatars, respectively. Figure 1: Schematic illustration of the dual-primate set-up. The master is displayed on top and the avatar is displayed on the bottom. Note that on decoding-based sessions, the master had a joystick during training that was then disconnected during the real-time neural prosthetic trials. On adaptive-based sessions, no joystick was used at any time. Under ‘empiric mapping’, the arrows indicate the estimated intended target of movement based on neural activity and the colour codes illustrate the corresponding stimulator channel used to elicit limb movement in the animal. The left versus right pairings indicate the two possible mappings to movement to each of the targets for the first and second avatars, respectively. Full size image During each session, the master was seated in a primate chair placed within a radiofrequency shielded recording enclosure. Simultaneous multiple-unit recordings were made from the master’s premotor cortex using chronically implanted planar multielectrode arrays (NeuroNexus Technologies Inc., MI). Signals were digitized and processed to extract action potentials in real-time by a Plexon workstation (Plexon Inc., TX). The avatar was fully sedated (using a combination of ketamine, xylazine and atropine) and was seated in a separate enclosure. The avatar’s limb was attached to a planar, free range-of-motion (360 degree), spring-loaded joystick that controlled a cursor displayed on the master’s screen. All trials during the task began with presentation of a small circular target that was positioned at two random locations on the screen. The radius of the targets displayed to the masters was 3.75 cm, with each target occupying ~8% of the screen surface at 24 cm × 24 cm. After presentation of a go cue, the master had to reach the displayed target by directing a cursor, from the centre of the screen to the displayed target, using stimulation-elicited limb movement in the avatar ( Fig. 2 ). The cursor had to occupy the target circumference for 100 ms or more in order for the master to receive reward (see Methods). 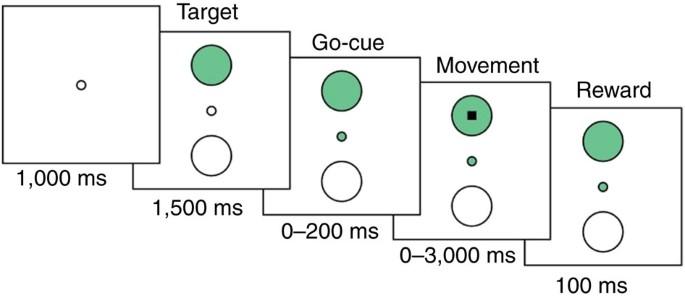Figure 2: Behavioural task. Schematic illustration of the trial presentation and timeline proceeding from left to right. On decoding-based sessions, a central green circle was used as a go cue. On adaptive, single-neuron based sessions, no go cue was given. Only the displayed target is shown on this particular trial (that is, the other possible target/movement locations are not shown). During model training and adaptive sessions, the monkeys had up to 3,000 ms to make a movement. Figure 2: Behavioural task. Schematic illustration of the trial presentation and timeline proceeding from left to right. On decoding-based sessions, a central green circle was used as a go cue. On adaptive, single-neuron based sessions, no go cue was given. Only the displayed target is shown on this particular trial (that is, the other possible target/movement locations are not shown). During model training and adaptive sessions, the monkeys had up to 3,000 ms to make a movement. Full size image Decoding intended movements using neural population activity We first used a population decoding approach that estimated the intended target of movement based on changes in the firing activity of neurons recorded within the master’s premotor cortex. Before performing the real-time neural prosthetic experiments, the spiking activity of all premotor neurons in the masters were modelled as an inhomogeneous Poisson process in a training session in which they used the joystick to perform the task [7] , [8] , [10] , [28] . This target-decoding approach is based on prior work by our group and others showing that multiple targets or target sequences can be accurately decoded from premotor neurons before movement (see Methods). We recorded a total of 125 well-isolated premotor neurons (11–20 units per session) over 10 sessions. To predict the planned movement before its execution, we analysed the neuronal activity during the target presentation period before the go cue. We find that, of the 125 cells recorded, 64 (51%; one-tailed Z -test, P <0.01; Fig. 3a ) significantly predicted which target the animals were intending to move to. When further examining model predictions based on the population activity at different time points, accuracy was 82±12% (mean±s.d.) by 500 ms after target presentation and 95±10% by 1,000 ms after target presentation across sessions consisting of 854 trials. By the time the go cue was first displayed, mean cross-validated prediction accuracy was 96±10% (one-tailed t -test, n =10; P <0.01; Fig. 3b ). Training across sessions was performed for an average of 85±19 trials (mean±s.d.) or ~6 min before performing the real-time experiments. 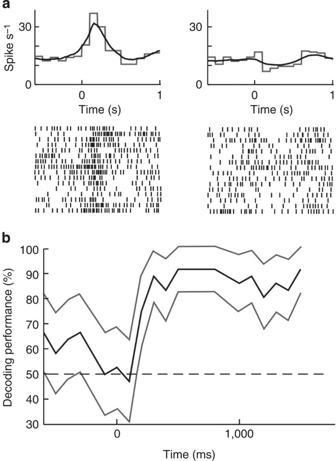Figure 3: Neural population decoding. (a) Averaged (grey) and model estimated (black) peristimulus histogram (top) and raster (bottom) of a premotor neuron during movement planning and aligned to presentation of two different targets (left and right, respectively). (b) Mean population decoding performance across all trials and 95% confidence bounds aligned to target presentation (and up to the go cue) during a sample session. Figure 3: Neural population decoding. ( a ) Averaged (grey) and model estimated (black) peristimulus histogram (top) and raster (bottom) of a premotor neuron during movement planning and aligned to presentation of two different targets (left and right, respectively). ( b ) Mean population decoding performance across all trials and 95% confidence bounds aligned to target presentation (and up to the go cue) during a sample session. Full size image Testing stimulation-elicited limb movements To elicit movement in the avatars, stimulating electrodes were chronically implanted in the cervical spinal cord of both monkeys. Two 16-contact iridium oxide stimulating electrodes (100–500 kΩ) were each inserted at the C5 and C6 levels of both avatars (NeuroNexus). In addition to spinal cord electrode implantation, percutaneous electrodes (100–200 kΩ) were placed in the long and short head of the triceps muscle of avatar #1. This was done to provide added range of movements not available by spinal cord stimulation in that particular avatar (see Methods for further discussion and Results). Before running the real-time combined recording-elicitation experiments, the stimulating electrodes were tested under different amplitudes and contact locations to determine the range of target locations that can be reached. Specifically, we identified which limb movement direction and amplitude will be produced per stimulation setting and contact location in the avatars and, therefore, to which precise target in space the cursor could reach. Similar to prior reported stimulation experiments in anesthetized animals [22] , [23] , [24] , [29] , [30] , [31] , we tested each contact location at serially incremented amplitudes. In all cases, stimulation frequency was 200 Hz and pulse width was 0.2 ms, with cathodal pulse leading. Stimulation duration was 500 ms and was selected to mimic the time it naturally took the masters to move to and hold a target during the normal joystick movement task (that is, non-prosthetic controlled). The tested stimulation amplitudes ranged from 10–80 μA and were incremented by 10–20 μA intervals per electrode contact. For both avatar 1 and 2, stimulations were tested across all 32 electrode contacts located within the ventral spinal cord at the C5–6 level (4-mm deep from the dorsal surface and 2-mm lateral from the median sulcus). For avatar 1, stimulations were also tested across four acute contacts located within the short and long head of the triceps muscle. In this case, stimulation frequency was 200 Hz and pulse width was 0.2 ms with cathodal pulse leading. Stimulation duration was 500 ms. The tested stimulation amplitudes ranged from 100–200 μA incremented by 10–20 μA intervals per electrode contact. We defined the targets of elicited movement based on the angle and amplitude of cursor displacement during the last 100 ms of stimulation. Here, the last 100 ms of stimulation was defined as the target ‘hold-time’ and was required in order for the master to receive reward. On average, each electrode array produced movements over a range of end target locations. These individual clusters ranged in width from ~6 to 7 cm. Triceps muscle stimulations were somewhat more confined, producing a cluster of end target locations 3.8-cm wide ( Fig. 4a,b ). 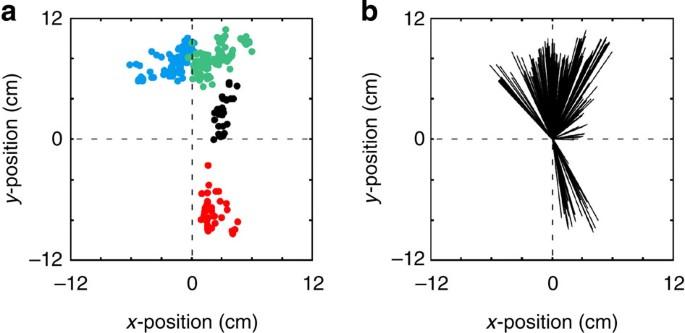Figure 4: Microstimulation-induced limb movement during testing. (a) Scatter plot indicating the mean cursor position during the last 100 ms of stimulation (during which the target was held) for all tested electrode sites. These together define the possible range of movements elicited in the two avatars during testing. For avatar #1, blue dots indicate the end targets of movement produced by C5 electrode stimulation and red dots indicate the end targets of movement produced by triceps stimulation. For avatar #2, green dots indicate the end targets of movement produced by C5 electrode stimulation and black dots indicate the end targets of movement produced by C6 stimulation. (b) Distribution of elicited movement directions in relation to centre. Figure 4: Microstimulation-induced limb movement during testing. ( a ) Scatter plot indicating the mean cursor position during the last 100 ms of stimulation (during which the target was held) for all tested electrode sites. These together define the possible range of movements elicited in the two avatars during testing. For avatar #1, blue dots indicate the end targets of movement produced by C5 electrode stimulation and red dots indicate the end targets of movement produced by triceps stimulation. For avatar #2, green dots indicate the end targets of movement produced by C5 electrode stimulation and black dots indicate the end targets of movement produced by C6 stimulation. ( b ) Distribution of elicited movement directions in relation to centre. Full size image Of the above tested contact locations and stimulation parameters, two were used for each session and avatar to produce stimulation-induced limb movements. These parameters were chosen to produce movements to targets that were distinct and as radially distant from each other as possible using the available implanted electrodes (in principal, however, and as discussed further below, any other stimulation parameters and corresponding elicited limb movements could be used for the task). The mean angle of separation between the two tested movements was 176 degrees for avatar #1 and 34 degrees for avatar #2 ( Fig. 5 ). For avatar #1, mean path length of movement was 10.3±0.2 cm and mean velocity was 86.4±9.0 cm s −1 (mean±s.d.). For avatar #2, mean path length of movement was 9.4±0.1 cm and the mean velocity was 59.6±3.0 cm s −1 . Mean deviation of movement (that is, how much the movement trajectory deviated from a straight line) was 1.0 cm for avatar #1 and 3.1 cm for avatar #2. 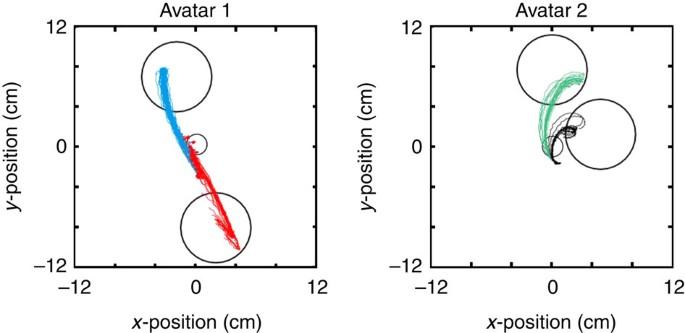Figure 5: Selected targets and elicited limb movement trajectories used for the real-time sessions. Target locations and the stimulation-induced limb movement trajectories are shown for avatar #1 (left) and avatar #2 (right). For avatar #1, upward movements (blue) were produced by C5 electrode stimulation and downward movements (red) by triceps stimulation. For avatar #2, upward movements (green) were produced by C5 electrode stimulation and righward movements (black) by C6 stimulation. Figure 5: Selected targets and elicited limb movement trajectories used for the real-time sessions. Target locations and the stimulation-induced limb movement trajectories are shown for avatar #1 (left) and avatar #2 (right). For avatar #1, upward movements (blue) were produced by C5 electrode stimulation and downward movements (red) by triceps stimulation. For avatar #2, upward movements (green) were produced by C5 electrode stimulation and righward movements (black) by C6 stimulation. Full size image Real-time neural prosthetic control of limb movement On the basis of the above testing, we could now predict the intended target of movement based on recorded premotor activity in the master and determine which spinal cord and/or muscle electrode locations and stimulation parameters elicit limb movement to the different targets positioned on the screen. Next, we approximated changes in motor intent with movement production using the master–avatar primates in real-time on a trial-by-trial basis. As the two targets were displayed in random order on the screen, neuronal activity was continuously recorded from the master and was used to predict trial-by-trial changes in the masters’ intended target of movement. Therefore, if neural activity recorded during the trial predicted that the master was intending to move to target #1, the system would activate the stimulating electrode in the avatar that was previously observed to produce limb movement to that exact target location. Alternatively, if neuronal activity predicted that the master was intending to move towards target #2, the system would activate another electrode that produced a movement towards that target. This way, the neural prosthesis continuously matched the master’s planned target of movement with stimulation parameters/electrode locations that elicited movement in the avatar’s limb to the same target. Importantly, selected stimulation parameters and electrode contacts were set to produce limb movement that precisely reached and held the intended target in their 2D space ( Fig. 1 ). As noted above, mean cross-validated performance during model training was 96±10% when tested across training sessions with 854 training trials ( Fig. 2b ). We find that, when the masters performed the same task as before but target selection was controlled by joystick movements made by the avatar using the neural prosthetic, performance was slightly lower but still significantly higher than chance. Overall, the primates reached the displayed targets during these real-time recording-elicitation sessions in 84±14% (mean±standard error of the mean (s.e.m.)) of the 561 trials tested (binomial test, P <0.01). Most incorrect trials (11%) occurred because of decoding error (that is, selecting the wrong target). Only a few errors (5%) occurred because the avatar-controlled cursor failed to reach the spatial confines of the displayed target (that is, to maintain the cursor location within the 0.75 radians or 8% screen surface of the target for 100 ms). No movements were made by the master during the decoding period, before the go cue presentation (that is, the trial would abort if any movement was made). To further confirm that no movements were made, we recorded electromyography (EMG) activity from the master as the task was being performed over one session (see Methods). We found no difference in activity during the decoding period, before the go cue, between planned movements ( t -test, P =0.53; Fig. 6 ). 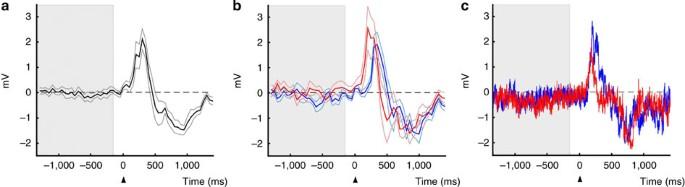Figure 6: EMG tracings display robust peri-movement activity during movement to both targets. (a) Averaged EMG tracings in millivolts over the course of a real-time recording-elicitation session. The grey area indicates the time during which neural decoding was performed and the arrow (time zero) indicates the time of the go cue. The thick line indicates the average activity and the thin lines the s.e.m. (b) EMG tracings are broken down into target of movement (red for up and blue for right). (c) Raw EMG tracings over two individual trials with the same colour convention as inb. Figure 6: EMG tracings display robust peri-movement activity during movement to both targets. ( a ) Averaged EMG tracings in millivolts over the course of a real-time recording-elicitation session. The grey area indicates the time during which neural decoding was performed and the arrow (time zero) indicates the time of the go cue. The thick line indicates the average activity and the thin lines the s.e.m. ( b ) EMG tracings are broken down into target of movement (red for up and blue for right). ( c ) Raw EMG tracings over two individual trials with the same colour convention as in b . Full size image Motor control based on adaptive sensorimotor responses In many circumstances, such as in the setting of full motor paralysis, it may not be possible to train models based on the subject’s natural movement. Also decoders trained on physical movement by the subjects may not accurately model the subjects’ planned movement during direct neural prosthetic control [32] , [33] , and consequently adaptive changes in neural activity may allow for improved performance over time. We tested this possibility by assigning individual neurons within the same premotor population (that is, the same recording electrodes) to control the avatar’s limb movement by volitionally modulating their activity. Similar to a sensorimotor conditioning approach described previously [21] , [34] , [35] , we randomly selected individual neurons and assigned them to control the target of movement by naturally varying their firing activity from trial to trial as the monkeys performed the same real-time neural prosthetic task above. In particular, depending on whether the firing activity of the assigned individual neuron went above or below a fixed firing rate threshold, movement would be elicited to one of the two targets (see Methods). Importantly, the mapping between the neuron’s firing activity and target location was chosen randomly, and no joystick was used by the master at any time ( Fig. 7a ). 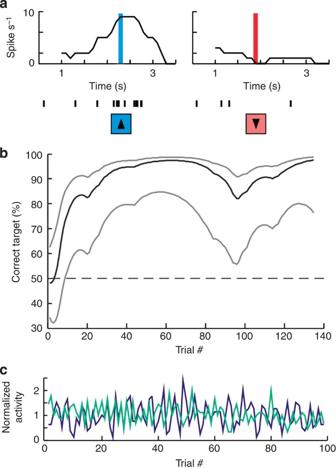Figure 7: Adaptive activity based approach for controlling movement. (a) The firing rate and corresponding spike time indicators (immediately blow thexaxis) of a single selected premotor neuron recorded over two individual trials aligned to target presentation for two different targets. The vertical bars indicate the time during which the firing rate of the neuron reached the top threshold (left, blue) and bottom threshold (right, red; see Methods for further detail on threshold definition). The arrows indicate the time of stimulation and mapped elicited limb movement for each trial. (b) Behavioural performance and 99% confidence bounds over successive trials witihin a session (100% performance indicates that the primates correctly selected and spatially reached the displayed target on all trials). (c) Example of the normalized firing activities (averaged firing rate within successive 1,000 ms windows divided by the mean firing rate across the entire session) of a selected (green) and a non-selected (purple) premotor neuron recorded over a single representative session. Figure 7: Adaptive activity based approach for controlling movement. ( a ) The firing rate and corresponding spike time indicators (immediately blow the x axis) of a single selected premotor neuron recorded over two individual trials aligned to target presentation for two different targets. The vertical bars indicate the time during which the firing rate of the neuron reached the top threshold (left, blue) and bottom threshold (right, red; see Methods for further detail on threshold definition). The arrows indicate the time of stimulation and mapped elicited limb movement for each trial. ( b ) Behavioural performance and 99% confidence bounds over successive trials witihin a session (100% performance indicates that the primates correctly selected and spatially reached the displayed target on all trials). ( c ) Example of the normalized firing activities (averaged firing rate within successive 1,000 ms windows divided by the mean firing rate across the entire session) of a selected (green) and a non-selected (purple) premotor neuron recorded over a single representative session. Full size image Using this approach, we recorded from 40 population cells. During these recordings, the primates performed 580 trials over five sessions. Starting performance by the selected cells was 37±10% (mean±s.e.m.) over the first 10 trials. Correct target selection, however, then rapidly improved, reaching an average performance of 77±12% (two-tailed t -test, n =5; P =0.02; Fig. 7b ). Overall, it took the monkeys 28±13 trials, or ~3 min, to reach statistical learning criterion (see Methods) [36] , [37] . The highest noted asymptotic performance was 90%. The mean firing rate of selected cells remained the same over the time course of these sessions when comparing the first and second half of the session (two-tailed t -test; P =0.88) as did variance in their firing rates (two-tailed t -test; P =0.92). During these adaptive sessions, no joystick was given to the monkeys and no visible movement was noted during the task. To further confirm that no subthreshold movements were being made, we recorded EMG activity from the master over one session. We found no change in EMG activity during selection of one target versus the other (area under the curve; two-tailed t -test, P =0.62) and no difference in EMG activity before versus after target presentation (windows=3,000 ms; two-tailed t -test, P =0.33; Fig. 8 ). 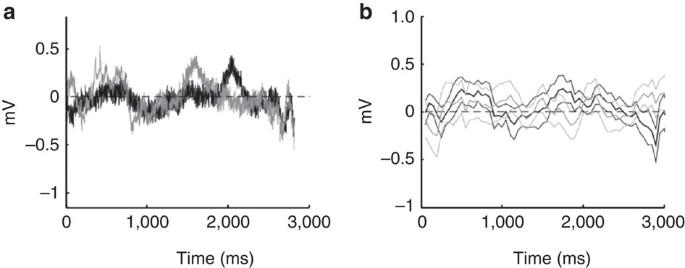Figure 8: EMG tracings in the master during the real-time adaptive recording-elicitation sessions. (a) An example of raw EMG tracings recorded in the master over individual trials during selection of the top (black) versus bottom (grey) target. In both trials, the window over which neuronal threshold was reached lied between 1,500–2,500 ms. (b) Average EMG activity for all top versus bottom movements over the course of the session, with the same colour convention as ina. The thick lines indicate the mean EMG activity in millivolts and the thin lines indicate their s.e.m. Figure 8: EMG tracings in the master during the real-time adaptive recording-elicitation sessions. ( a ) An example of raw EMG tracings recorded in the master over individual trials during selection of the top (black) versus bottom (grey) target. In both trials, the window over which neuronal threshold was reached lied between 1,500–2,500 ms. ( b ) Average EMG activity for all top versus bottom movements over the course of the session, with the same colour convention as in a . The thick lines indicate the mean EMG activity in millivolts and the thin lines indicate their s.e.m. Full size image Response of non-selected neurons during adaptive control Since each selected neuron can only encode a binary response using this potential approach (that is, high versus low threshold), we wanted to determine whether other neurons not involved in controlling movement respond similarly to the intended targets. This may, therefore, provide insight into the potential capacity of larger neural populations and distinct selected cells to adaptively direct movement to more than two targets at a time. By simultaneously recording from multiple neurons during these sessions, we found that neighbouring neurons in the premotor population displayed surprisingly little correspondence with the activities of the selected neurons. Thirty five premotor cells were recorded over the same five sessions in addition to the selected cells. However, none of the recorded cells demonstrated a significant correlation (either positive or negative) when comparing the time-varying firing rates of selected cells to the other non-selected cells (Pearson’s correlation, n =35; P >0.05). In other words, cells that were not selected to control movement did not consistently increase their firing activity when the activity of the selected cell increased during targeted movement or vice versa (note that these single cells were selected randomly from the population and the mapping between their firing rates and target selection was chosen arbitrarily). An example of two such cells is shown in Fig. 7c (also, note that both cells still markedly fluctuated their activities from trial to trial). Similarly, there was little correlation in activity when considering variations in the firing activities across all pairings (mean correlation r =−0.012±0.022; mean±s.e.m.). These findings, therefore, suggested that cells in the population not directly assigned to controlling the movement do not necessarily covary their activities with the intended target during artificial motor control. Achieving volitional control of one’s own limb has been an important goal in the field of neural prosthetic development. Recent work has shown that the intended targets of movement or movement sequences can be inferred from primary motor and premotor neurons and that, even with a small number of recorded cells, it is possible to distinguish between multiple distinct planned targets in space [8] , [10] , [28] . On the basis of this initial evidence, the basic question that we aimed to investigate was whether it is possible to couple, in real-time, the animal’s intended target of movement with unconstrained (360 degree range of movement), stimulation-elicited limb movements to the same target confines in 2D space and under full functional paralysis. While such a goal will require continued technical innovation, as an initial proof of concept, we devised and tested a cortical–spinal neural prosthesis designed for controlling limb movements to two different small targets randomly positioned on a screen. We hypothesized that by focusing on the target of movement, rather than the ongoing planned trajectory, it may be possible to provide a simple solution for directing naturalistic limb movement to different targets in space. Prior work has tackled the problem of controlling limb movement by inferring the ongoing planned trajectory of movement in real time [20] . While this approach demonstrated the remarkable ability to elicit movement over a given trajectory, it is presently limited to directing movement to a single, repeated target in space. Hence the applicability of such an approach to generating movement towards distinct targets is unclear. Here, using an alternate approach that allows the animal to control only the intended target locations of movement, we show that it is possible to produce unconstrained limb movements to more than one precisely positioned target on a screen. While a range of angles and amplitudes of movements could be produced with only a few implanted spinal cord and muscle electrodes, it is likely that a larger number of electrodes and/or contact sites would be needed to allow for elicited movement to more than two targets. An obvious limitation, however, is that such an approach would not accurately mimic the precise intended trajectory of movement, which may also be important under certain task settings [7] , [19] . We also examined whether neurons, randomly selected from the population, could similarly control limb movement by volitionally modulating their activity, thus resulting in adaptive motor prosthetic control. To allow for comparison with the above decoding approach, we recorded from the same premotor microelectrodes and tested the same two target locations using the same task. We find that under this two-target setting, the animals learned to significantly improve the target acquisition accuracy over a fairly short time-period and were able to reach accuracies comparable to (albeit somewhat lower than) the decoding-based approach. Using this adaptive approach, we also examined how other non-selected neurons concomitantly changed their firing activities. Prior studies have demonstrated broad motor population responses to upcoming movements [1] , [2] , [3] , [38] , indicating that such neurons encode planned/intended movements as a concerted population-wide vector or function. A more recent important study has also shown that, when decoders were trained on the directional tuning of motor populations (that is, using multiple neurons), neurons that were not directly involved in prosthetic control continued to modulate with the animal’s movements but did so more weakly [39] . In agreement with these findings, we observe that individual neurons in the premotor cortex that are assigned to control the movement progressively modulated their activity with the intended targets. However, we also find that when motor control was assigned to individual neurons whose activity was mapped to movement arbitrarily, other surrounding cells did not consistently modulate their activity with the intended targets. While we used only a limited number of neurons recorded from small premotor populations, this finding suggests that it may be possible to orthogonally train more than one, and potentially multiple, single neurons to encode a different set of target locations. Therefore, either decoding- or adaptive-based approaches may be viable options for controlling such a target-based neural prosthetic and may provide straight forward means for artificially generating goal-directed movements under direct cortical control. Finally, to provide a model of paralysis in which to test present and future neural prosthetic approaches aimed at enabling limb movement in full paralysis, we introduced a novel two-primate set-up for functionally paralysing awake-behaving animals. This new technique was useful in that it provided a relatively simple way by which to dissociate all spinal cord pathways, and by which to test motor control without the influence of partially or completely preserved efferent/afferent circuitries [40] . Recent studies, in particular, have demonstrated that providing proprioceptive and kinesthetic feedback to healthy subjects performing a BMI task can significantly improve the BMI accuracy. Such feedback, however, is lost in paralysis and cannot help BMI performance in paralysed subjects [26] , [27] . This lack of proprioceptive feedback has been achieved in BMIs for control of external devices by partially restraining the animal’s arm [33] . However, in neural prosthetics aimed at controlling the limb, such an approach would not be possible and hence the two-primate set-up can provide a useful model by which to test such neural prosthetics. An analogous approach for using the nervous system of one animal to control the nervous system of another has also recently been employed to relay motor commands and sensory-related information [41] , [42] . A limitation of the dual-monkey model is that the monkeys do not display all the same clinical features as truly chronically paralysed animals such as muscle rigidity or autonomic dysreflexia [43] . However, and perhaps as importantly, paralysis was reversible and was not associated with the extreme morbidity inherent to spinal cord paralysis. Dual-primate spinal cord paralysis model Two adult male Rhesus macaques, ages 6–8-years old, were included in this study in accordance with IACUC guidelines and approved by the Massachusetts General Hospital institutional review board. Two monkeys were used to confirm reproducibility of results and neural–prosthesis performance. Each monkey, alternating in role for each session, acted either as the master or avatar. Here, the master was seated in a primate chair placed within a radiofrequency shielded recording enclosure (Crist Instrument Co. Ltd, Damascus, MD). The masters’ head was restrained using a head post, and a spout was placed in front of its mouth to deliver juice using an automated solenoid. A computer monitor that displayed the task was placed at eye level in front of the master. The primate acting as the avatar was seated in a separate enclosure. Its upper limb was secured onto a 360 degree, free range-of-motion, spring-loaded, joystick that controlled a cursor displayed on the master’s screen. A NI DAQ card (National Instruments, TX) was used for the I/O behavioural interface, and the behavioural programme was run in Matlab (MathWorks, MA) using custom made software routines [44] . On separate weeks, the two primates interchangeably acted as either the master or avatar. Therefore, if the primate was an avatar on a given week, we would use stimulation parameters and electrode locations specific to that monkey. Note that stimulation parameters that were previously demonstrated, during testing, to produce upward arm movement in avatar #1 may be different from parameters used in avatar #2. Recording multielectrode implantation Multiple recording silicone multielectrode arrays (NeuroNexus Technologies Inc., MI) were chronically implanted in each monkey [45] . A craniotomy was performed along the dorsal-lateral region of frontal lobe under standard stereotactic guidance (David Kopf Instruments, CA). After directly visualizing the cortical gyral pattern underlying the craniotomy, the arrays were implanted into the dorsal and medial aspects of the premotor cortex (Brodmann area 6). This area was implanted with 3–4 arrays in each monkey, with each array possessing 32 electrode contacts in a 4 × 8 configuration. Spacing between vertical contacts was 200 μm and horizontal contacts 400 μm. Recordings began 2 weeks following surgical recovery. A Plexon multichannel acquisition processor was used to amplify and band-pass filter the neuronal signals (150 Hz–8 kHz; 1 pole low-cut and 3 pole high-cut with 1,000 × gain; Plexon Inc., TX). Signals were digitized at 40 kHz and processed to extract action potentials in real-time by the Plexon workstation. Classification of the action potential waveforms was performed using template matching and principle component analysis based on waveform parameters. Only single, well-isolated units with identifiable waveform shapes and adequate refractory periods were used for the online experiments and off-line analysis. No multiunit activity was used. For EMG recordings, we used tin surface electrodes from over the deltoid contralateral to neural recordings (this muscle displayed the most robust peri-movement activity during movement to both targets). Signals were digitized at 1 kHz and were recorded by the Plexon workstation. Stimulating electrode implantation Stimulating electrodes were chronically implanted in the cervical spinal cord of both monkeys. A dorsal skin incision was placed over the C5–6 lamina, and a laminectomy was performed to expose the dorsal spinal canal. In both avatars, two 16-contact iridium oxide stimulating electrode (100–500 kΩ) were inserted at the C5 and C6 levels (NeuroNexus Technologies Inc., MI). These were placed to a depth of 4 mm from the dorsal surface and 2 mm lateral from midline, corresponding to the approximate location of the ventral horn of the spinal cord. A fibrin sealant (Baxter, IL) was used to cover the dural opening, and the distal female connector was secured into place using a titanium mini-plate and acrylic cement along the lateral laminar edge. In addition to spinal cord electrode implantation, percutaneous electrodes (100–200 kΩ) were each placed, under sterile preparation, in the long and short head of the triceps muscle of avatar #1. The connecting wires were secured into place using an elastic cuff and attached to a female connector. Behavioural task All trials during the task began with presentation of a circular green target that was randomly positioned in one of two locations on a screen (roughly, top versus bottom of the screen during avatar #1 sessions and top versus right of the screen during avatar #2 sessions). On decoding-based sessions, a go cue would appear 1,500 ms after target onset, following which time the master was allowed to move the joystick to guide a cursor from the centre of the screen to the intended target. During real-time performance of the recording-elicitation sessions, the exact same sequence of target presentations and go cue timings would be given but, now, movement of the cursor would be based on joystick-attached limb movements made by the avatar. The master only received reward if the displayed target was reached and held for 100 ms. Target selection based on decoded population responses We first inferred the planned target of movement in the master based on neural activities recorded in their premotor cortex. Using a population decoding approach, we determined the intended target of movement based on the firing activities of the neuronal population as masters performed the task. To estimate the masters’ planned target of movement, we initially trained the models on the activity of neuronal populations in their premotor cortex as they performed the task using a joystick during the training sessions. The spiking activity of each neuron was modelled as an inhomogeneous Poisson process whose likelihood function is given by where Δ is the time increment taken to be small enough to contain at most one spike, is the binary spike event of the c th neuron in the time interval (( k −1)Δ, k Δ), λ c ( k | S i ) is its instantaneous firing rate in that interval, S i is the i th target of movement, and K is the total number of bins in a duration K Δ. We take Δ=5 ms as the bin width of the spikes. For each target and neuron, we estimated the firing rate λ c ( k | S i ) over the 1,500 ms target presentation period (before the go cue) using a state-space expectation-maximization approach [28] . After fitting the models, we validated them using the χ 2 goodness-of-fit test on the data and confirmed that they fitted the data well ( P >0.7 for all cells in all sessions). As noted in the main text, we had previously used such a decoding approach to infer the intended target of movement of primates across multiple targets and target sequences (that is, up to 12). For the purpose of the present experiments, we decoded only two targets at a time. During real-time recording-elicitation neural prosthetic experiments, the master’s joystick was disconnected and the intended target of movement was inferred using a maximum-likelihood decoder based on neuronal activity recorded from the same premotor population. The maximum-likelihood decoder was used to determine the intended target based on the neuronal activity recorded over 1,500 ms during the target presentation period and before the animals movement [28] . Using the model above, the population likelihood under any target is given by where K is the total number of bins (300) during the target presentation period, C is the total number of neurons, and λ c ( k | S i ) for k =1, …, K and c =1, …, C is the estimate of the firing rate. The decoded target was selected as the one that had the highest population likelihood. Finally, we evaluated the accuracy of the decoders obtained during the training session using leave-one-out cross-validation. This allowed us to examine the accuracy of the trained models on a trial-by-trial basis. Threshold and target determination on adaptive sessions In a separate set of sessions, single neurons were individually selected from the same premotor population (that is, recording electrode contacts) in the master and were randomly assigned to control limb movement produced by the avatar. These selected neurons were allowed to naturally vary their firing activity from trial to trial and, depending on whether their firing activity went above or below a fixed firing rate threshold, movement to one of the two possible target locations would be elicited. Importantly, the mapping between the neuron’s firing activity, target location and elicited movement was chosen randomly. Moreover, unlike the decoding-based approach, no joystick was used by the master at any time [46] . With regards to determining the thresholds, before performing the recording-elicitation sessions, the natural firing rate distribution of the selected neuron was determined by recording its spiking activities while the master remained at rest for 5 min. Following this, the top 90th and bottom 10th percentiles of that distribution were determined. Each threshold was randomly assigned to correspond to selection of movement to one of the two displayed targets (for example, reaching the low threshold could correspond to movement to the top target whereas reaching a high threshold could correspond to movement to the bottom target, or vice versa, on a given session). On each trial during the real-time recording-elicitation sessions, the firing rate of the same selected neuron would be calculated in 1,000 ms windows advanced in 100 ms increments (that is, total number of spikes counted over 1 s). If at any point after an initial 1,500 ms delay the firing rate of the selected neuron reached either the top 90th or the bottom 10th percentile of their firing rate distribution, one of the two possible targeted movements would be elicited in the avatar. Reward would only be given to the master if the correct displayed target was reached and held for 100 ms (note that, since a target would be selected if either threshold was reached within a 1,500 ms trial duration, there was only a 0.8 15 chance that no movement would be elicited, meaning that movement was elicited in essentially all trials). Statistical testing Correlated activity between selected and other non-selected neurons within the recorded premotor population was assessed based on their Pearson’s product-moment coefficients ( P< 0.05). Evaluating accuracy of behavioural performance above chance was assessed using a binomial test ( P <0.05), and change in performance across sessions was assessed by a two-tailed t -test ( P <0.05). All these values were given with their s.e.m.. Behavioural performance was estimated from the animals’ binary responses (correct versus incorrect target) using a Bernoulli state-space approach described previously [36] , [37] . Briefly, this was accomplished by fitting the curve to a standard logistic equation, which provided a continuous estimate, ranging from 0 to 1, of the animals’ learning performance. The 99% confidence bounds of the curve were used to determine when learning criterion was statistically achieved (that is, when the confidence bounds first went above 50% chance). With regards to kinematics, the displacement and velocity of movements were calculated from the trajectory tracings of each movement. The standard deviation of movement was determined by calculating the distance between each point along the trajectory of the cursor (that is, as it curvilinearly moved from the centre of the screen to the target) and that of the optimal trajectory (that is, a straight line from the centre of the screen to the centre of the displayed target). How to cite this article: Shanechi, M. M. et al. A cortical–spinal prosthesis for targeted limb movement in paralysed primate avatars. Nat. Commun. 5:3237 doi: 10.1038/ncomms4237 (2014).